PHD3 regulates EGFR internalization and signalling in tumours Tumours exploit their hypoxic microenvironment to induce a more aggressive phenotype, while curtailing the growth-inhibitory effects of hypoxia through mechanisms that are poorly understood. The prolyl hydroxylase PHD3 is regulated by hypoxia and plays an important role in tumour progression. Here we identify PHD3 as a central regulator of epidermal growth factor receptor (EGFR) activity through the control of EGFR internalization to restrain tumour growth. PHD3 controls EGFR activity by acting as a scaffolding protein that associates with the endocytic adaptor Eps15 and promotes the internalization of EGFR. In consequence, loss of PHD3 in tumour cells suppresses EGFR internalization and hyperactivates EGFR signalling to enhance cell proliferation and survival. Our findings reveal that PHD3 inactivation provides a novel route of EGFR activation to sustain proliferative signalling in the hypoxic microenvironment. Sustained proliferative signalling is a central hallmark of cancer, which allows tumour cells to overcome growth limitations and proliferate continuously within the tumour microenvironment [1] . These aberrant growth characteristics can be attributed to the deregulation in the signalling cascade of a number of growth factors and their receptors (reviewed in ref. 2 ). In particular, unrestrained activation of epidermal growth factor receptor (EGFR) signalling is a common feature in the pathology of many malignant tumours, including malignant glioma [3] . Ligand-induced activation of EGFR and subsequent tyrosine phosphorylation at the cytoplasmic tail leads to the recruitment of proteins that ultimately downregulates EGFR signalling through endocytosis [4] , [5] . Unrestrained tumour growth is commonly associated with a hypoxic tumour microenvironment, as highly proliferating tumours frequently outstrip their vascular supply. Hypoxia initiates multiple cellular responses, primarily through the hypoxia-inducible factors (HIFs) [6] , which allow tumour cells to promote their growth and progression towards a more malignant phenotype. In most cell types, a decrease in cellular proliferation or even cell cycle arrest is hardwired into the program of oxygen conformance as a fundamental physiological response to hypoxia [7] , [8] to enable cell survival through depression of the cellular metabolism [9] . Little is known about how tumours sustain proliferative signalling and counteract the growth-suppressing effects of the hypoxic microenvironment. The prolyl hydroxylase domain proteins 1–3 (PHDs; also called EglN) [10] , [11] have been identified as key regulators of HIFs [12] . In addition, PHDs also possess important HIF-independent functions [13] , [14] , [15] , [16] , [17] , [18] . A growing body of evidence underlines the importance of PHDs in tumour progression. Tumour-promoting and -inhibiting functions have been described for PHD1 (refs 19 , 20 ) and PHD2 (refs 13 , 21 , 22 ), whereas several recent reports highlight a tumour-suppressive role of PHD3 in several types of cancer [18] , [23] , [24] , [25] . As PHD3 is strongly regulated by hypoxia and other stress-related mechanisms [26] , [27] , PHD3 may act as a key sensor of stress signals within the tumour microenvironment. Here we were interested to mechanistically understand how PHD3 regulates tumour growth in response to microenvironmental signals. PHD3 loss sustains proliferation through EGFR activation We have identified PHD3 as a key regulator of tumour growth in response to hypoxia and showed that loss of PHD3 resulted in increased EGFR phosphorylation [28] . As the hyperactivation of EGFR signalling has a central role in malignant transformation in gliomas [3] , we next investigated whether the growth advantage following PHD3 loss could be the result of a deregulated EGFR function due to a molecular crosstalk between PHD3 and EGFR signalling. G55 glioblastoma cells with a lentiviral knockdown of PHD3 exhibited a striking and prolonged increase in EGFR phosphorylation ( Fig. 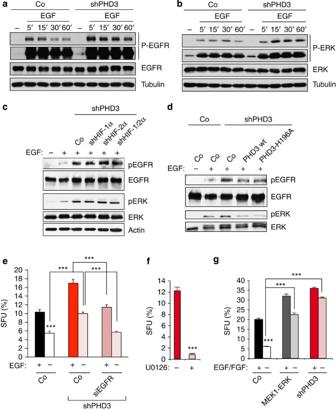Figure 1: Loss of PHD3 enhances EGFR signalling. (a,b) PHD3 loss enhances EGFR phosphorylation (a) and signalling (b). Immunoblot of (P-)EGFR (a) and (P-)ERK (b) of G55 cells expressing control or PHD3 shRNA that were non-stimulated or EGF stimulated for the indicated times. (c) Enhanced EGFR signalling following PHD3 loss is HIF-1/2α independent. Immunoblot of (P-)EGFR and (P-)ERK of G55 cells expressing control or PHD3 shRNA in combination with control, HIF-1α or HIF-2α or double HIF-1α/2α shRNA that were non-stimulated or EGF stimulated for 5 min. (d) Immunoblot of (P-)EGFR and (P-)ERK of G55 cells expressing control or PHD3 shRNA that were transfected with wild-type PHD3, the hydroxylase mutant PHD3-H196A or empty vector control and were non-stimulated or EGF stimulated for 5 min. (e) EGFR mediates the growth-promoting effect of PHD3 loss. G55 cells expressing control or PHD3 shRNA were cultured as spheroids in B27-supplemented serum-free medium±EGF (20 ng ml−1) and transfected with control or EGFR siRNA. The number of spheroids was quantified after 3 days (n=6). (f) MAPK signalling is required for the growth-promoting effect of PHD3 loss. G55 tumour cells expressing PHD3 shRNA were cultured as spheroids in B27-supplemented serum-free medium without growth factors±treatment with the MAPK inhibitor U0126 (10 μM) and the number of spheroids was quantified after 3 days (n=6). (g) Constitutively active MAPK signalling phenocopies PHD3 deficiency. G55 cells expressing control or PHD3 shRNA were transfected with a constitutively active MAPK construct (MEK1-ERK) or control vector, cultured as spheroids in B27-supplemented serum-free medium±EGF/FGF and the number of spheroids was quantified after 3 days (n=6). Western blot images (a–d) have been cropped for presentation. Full-size images are presented inSupplementary Fig. 5. All values are means+s.e.m., Student’st-test ***P<0.001. 1a ; Supplementary Fig 1a ). Moreover, PHD3 loss enhanced mitogen-activated protein kinase (MAPK) signalling as evidenced by increased ERK1/2 phosphorylation ( Fig. 1b ; Supplementary Fig. 1b ) and activated transcriptional responses downstream of MAPK as evidenced by increased SRE (serum response element) promoter reporter activity ( Supplementary Fig. 1c ). These results were confirmed using a different short hairpin RNA (shRNA) sequence targeting PHD3 in G55 cells ( Supplementary Fig. 1d ), as well as in the PHD3-silenced primary glioblastoma cell line GBM046x ( Supplementary Fig. 1e ) and in murine high-grade astrocytoma cells lacking PHD3 (PHD3 −/− astrocytomas [28] ; Supplementary Fig. 1f ). Importantly, the increased EGFR phosphorylation after PHD3 loss was not abolished by silencing of HIF1α and/or HIF2α ( Fig. 1c ) and was partially rescued by both the wild-type and a hydroxylase-deficient H196A PHD3 mutant ( Fig. 1d ). These findings are in agreement with a function of PHD3 in tumour growth control independent of HIF and of its hydroxylase activity [28] . Notably, the control of EGFR signalling was specific for the PHD3 isoform since loss of PHD2 did not significantly alter EGFR phosphorylation ( Supplementary Fig. 1g ), which is in line with the PHD3 (and not PHD2)-dependent control of tumour growth observed in glioblastomas [28] . Therefore, our results show that PHD3 disruption potently activates EGFR signalling. We next investigated whether the growth-promoting effects of PHD3 inactivation are functionally dependent on the increased EGFR signalling. To this end, we used a functional in vitro assay employing a three-dimensional tumour spheroid culture system under defined serum-independent conditions that more closely replicates the growth characteristics of tumours in vivo . PHD3 loss prominently increased the number of spheres as a parameter of clonal outgrowth and EGFR silencing reversed the growth-promoting effect of PHD3 disruption ( Fig. 1e ). Moreover, inhibition of downstream signalling using the MAPK inhibitor U0126 abrogated growth following PHD3 loss ( Fig. 1f ). Conversely, a constitutively active MAPK mutant mimicked the effect of PHD3 loss ( Fig. 1g ). These results confirm that sustained proliferative signalling on PHD3 loss is the result of increased EGFR activation. Taken together, our results identify PHD3 as a potent regulator of EGFR signalling and reveal a novel route of EGFR activation in tumours. Figure 1: Loss of PHD3 enhances EGFR signalling. ( a , b ) PHD3 loss enhances EGFR phosphorylation ( a ) and signalling ( b ). Immunoblot of (P-)EGFR ( a ) and (P-)ERK ( b ) of G55 cells expressing control or PHD3 shRNA that were non-stimulated or EGF stimulated for the indicated times. ( c ) Enhanced EGFR signalling following PHD3 loss is HIF-1/2α independent. Immunoblot of (P-)EGFR and (P-)ERK of G55 cells expressing control or PHD3 shRNA in combination with control, HIF-1α or HIF-2α or double HIF-1α/2α shRNA that were non-stimulated or EGF stimulated for 5 min. ( d ) Immunoblot of (P-)EGFR and (P-)ERK of G55 cells expressing control or PHD3 shRNA that were transfected with wild-type PHD3, the hydroxylase mutant PHD3-H196A or empty vector control and were non-stimulated or EGF stimulated for 5 min. ( e ) EGFR mediates the growth-promoting effect of PHD3 loss. G55 cells expressing control or PHD3 shRNA were cultured as spheroids in B27-supplemented serum-free medium±EGF (20 ng ml −1 ) and transfected with control or EGFR siRNA. The number of spheroids was quantified after 3 days ( n =6). ( f ) MAPK signalling is required for the growth-promoting effect of PHD3 loss. G55 tumour cells expressing PHD3 shRNA were cultured as spheroids in B27-supplemented serum-free medium without growth factors±treatment with the MAPK inhibitor U0126 (10 μM) and the number of spheroids was quantified after 3 days ( n =6). ( g ) Constitutively active MAPK signalling phenocopies PHD3 deficiency. G55 cells expressing control or PHD3 shRNA were transfected with a constitutively active MAPK construct (MEK1-ERK) or control vector, cultured as spheroids in B27-supplemented serum-free medium±EGF/FGF and the number of spheroids was quantified after 3 days ( n =6). Western blot images ( a – d ) have been cropped for presentation. Full-size images are presented in Supplementary Fig. 5 . All values are means+s.e.m., Student’s t -test *** P <0.001. Full size image PHD3 interacts with EGFR and regulates its internalization To mechanistically address how PHD3 can control EGFR phosphorylation, we first confirmed that both proteins physically interact. Proximity ligation assays revealed that endogenous PHD3 and EGFR interact and that their physical interaction is enhanced by EGF and by hypoxia ( Fig. 2a ). Co-immunoprecipitation using G55 cells stably expressing a V5-tagged PHD3 confirmed that PHD3 interacts with EGFR ( Fig. 2b ; Supplementary Fig. 2 ) and that the interaction is enhanced following EGF stimulation ( Fig. 2c ). The signalling properties of EGFR are tightly controlled by its intracellular localization. Growth factor binding to EGFR activates receptor signalling and initiates a complex cascade that results in receptor inactivation by stimulating its endocytosis, followed by lysosomal targeting and degradation of internalized receptors [4] , [5] . We therefore assessed whether PHD3 controls EGFR activity by regulating the kinetics of its internalization. In line with a PHD3-dependent control of EGFR mobilization, we observed co-localization of PHD3 and EGFR in the early endosomal compartment ( Fig. 2d ). In control cells, EGFR was rapidly internalized following EGF treatment and localized to EEA1-positive early endosomes, peaking at 15 min ( Fig. 3a,b ). Starting at around 30 min after EGF stimulation, EGFR was transferred to M6PR-positive late endosomes ( Fig. 3c,d ). PHD3 loss abrogated this process and resulted in cell surface trapping of EGFR ( Fig. 3a–d ). Moreover, we confirmed these results biochemically by using a cell surface biotinylation capture enzyme-linked immunosorbent assay (ELISA). Loss of PHD3 impaired EGFR internalization as early as 2 min following stimulation with EGF ( Fig. 3e,f ; Supplementary Fig. 3a ). These findings were also corroborated by fluorescence-activated cell sorting (FACS) analysis of EGFR levels at the surface of control and EGF-stimulated glioma cells. Control cells exhibited a pronounced loss of surface EGFR signal at 15 min following EGF-induced EGFR internalization, whereas PHD3-deficient tumour cells largely retained EGFR at the cell surface ( Supplementary Fig. 3b,c ). Together, these results demonstrate that loss of PHD3 impairs EGFR internalization, suggesting that impairment of internalization underlies the enhanced EGFR signalling we observe in PHD3-depleted cells. To directly confirm that inhibition of internalization induces EGFR activation, we treated cells with dynasore, an inhibitor of dynamin-dependent endocytosis. Dynasore treatment resulted in retention of EGFR at the cell surface ( Fig. 4a,b ), similar to the one obtained following loss of PHD3 ( Fig. 3a–d ). Importantly, in both dynasore-treated and PHD3-deficient cells, this trapping of EGFR at the surface resulted in increased EGFR phosphorylation and signalling ( Figs 1a,b and 4c ). Thus, our findings indicate that PHD3 is required for EGF-induced EGFR internalization and that lack of PHD3 hyperactivates EGFR by inhibiting its endocytosis. 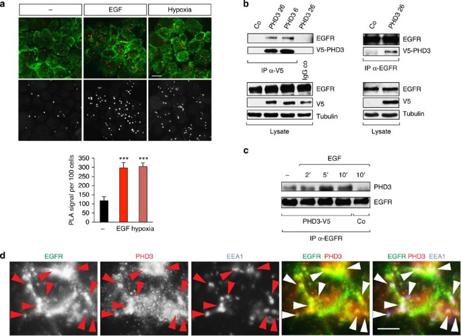Figure 2: PHD3 interacts with EGFR. (a) Interaction of endogenous EGFR and PHD3. Proximity ligation assay in G55 cells non-stimulated or stimulated for 5 min with EGF (20 ng ml−1) or exposed to 1% O2(hypoxia, 48 h). Red spots are sites of proximity ligation assay amplification reflecting the interaction between EGFR and PHD3, which is enhanced after EGF and hypoxia treatment. (b) Co-immunoprecipitation assay using anti-V5 or anti-EGFR antibodies and extracts from G55 cells expressing PHD3-V5 or GFP control, demonstrating interaction between PHD3 and EGFR. (c) The interaction between EGFR and PHD3 is induced by EGF. Co-immunoprecipitation assay using anti-EGFR antibodies from extracts of G55 cells expressing PHD3-V5 or GFP control and western blot of PHD3 and EGFR. Cells were non-stimulated or stimulated with EGF (20 ng ml−1) for the indicated times. (d) PHD3 co-localizes with EGFR at the plasma membrane and in the early endosomal compartment. Triple co-localization analysis of EGFR, PHD3 and the early endosomal compartment marker EEA1 in G55 cells expressing PHD3 stimulated for 5 min with EGF (20 ng ml−1). Arrows point to sites of triple co-localization. Western blot images (b,c) have been cropped for presentation. Full-size images are presented inSupplementary Fig. 6. All values are means+s.e.m., Student’st-test ***P<0.001. Scale bars, 10 μm (a), 5 μm (d). Figure 2: PHD3 interacts with EGFR. ( a ) Interaction of endogenous EGFR and PHD3. Proximity ligation assay in G55 cells non-stimulated or stimulated for 5 min with EGF (20 ng ml −1 ) or exposed to 1% O 2 (hypoxia, 48 h). Red spots are sites of proximity ligation assay amplification reflecting the interaction between EGFR and PHD3, which is enhanced after EGF and hypoxia treatment. ( b ) Co-immunoprecipitation assay using anti-V5 or anti-EGFR antibodies and extracts from G55 cells expressing PHD3-V5 or GFP control, demonstrating interaction between PHD3 and EGFR. ( c ) The interaction between EGFR and PHD3 is induced by EGF. Co-immunoprecipitation assay using anti-EGFR antibodies from extracts of G55 cells expressing PHD3-V5 or GFP control and western blot of PHD3 and EGFR. Cells were non-stimulated or stimulated with EGF (20 ng ml −1 ) for the indicated times. ( d ) PHD3 co-localizes with EGFR at the plasma membrane and in the early endosomal compartment. Triple co-localization analysis of EGFR, PHD3 and the early endosomal compartment marker EEA1 in G55 cells expressing PHD3 stimulated for 5 min with EGF (20 ng ml −1 ). Arrows point to sites of triple co-localization. Western blot images ( b , c ) have been cropped for presentation. Full-size images are presented in Supplementary Fig. 6 . All values are means+s.e.m., Student’s t -test *** P <0.001. Scale bars, 10 μm ( a ), 5 μm ( d ). 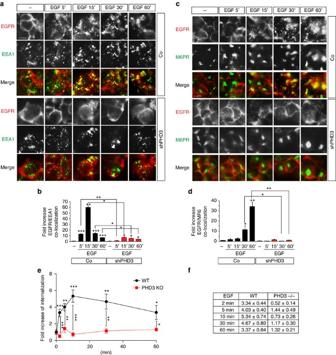Figure 3: Loss of PHD3 inhibits EGFR internalization. (a–d) EGFR internalization is inhibited on PHD3 loss. Immunofluorescence of G55 cells expressing control or PHD3 shRNA, non-stimulated or stimulated with EGF (20 ng ml−1) for the indicated times. EGFR co-localizes at early time points with EEA1, peaking at 15 min after stimulation (a,b). At later time points (30 and 60 min) after stimulation, EGFR co-localizes with the late endosomal marker mannose 6-phosphate receptor (M6PR;c,d). PHD3 loss compromises EGFR internalization, with EGFR remaining at the plasma membrane (a,c). The graphs show quantification of the increase in EGFR/EEA1 co-localization (b) and EGFR/M6PR co-localization (d) relative to non-stimulated cells (n=50–200). (e,f) Deletion of PHD3 blocks EGFR internalization. Internalization of EGFR in wild-type or PHD3−/− astrocytomas was quantitatively assessed by capture ELISA (n=6). The mean±s.e.m. is shown in the graph (e) and the table (f). All values are means+s.e.m., Student’st-test *P<0.05; **P<0.01; ***P<0.001. Scale bars, 10 μm. Full size image Figure 3: Loss of PHD3 inhibits EGFR internalization. ( a – d ) EGFR internalization is inhibited on PHD3 loss. Immunofluorescence of G55 cells expressing control or PHD3 shRNA, non-stimulated or stimulated with EGF (20 ng ml −1 ) for the indicated times. EGFR co-localizes at early time points with EEA1, peaking at 15 min after stimulation ( a , b ). At later time points (30 and 60 min) after stimulation, EGFR co-localizes with the late endosomal marker mannose 6-phosphate receptor (M6PR; c , d ). PHD3 loss compromises EGFR internalization, with EGFR remaining at the plasma membrane ( a , c ). The graphs show quantification of the increase in EGFR/EEA1 co-localization ( b ) and EGFR/M6PR co-localization ( d ) relative to non-stimulated cells ( n =50–200). ( e , f ) Deletion of PHD3 blocks EGFR internalization. Internalization of EGFR in wild-type or PHD3−/− astrocytomas was quantitatively assessed by capture ELISA ( n =6). The mean±s.e.m. is shown in the graph ( e ) and the table ( f ). All values are means+s.e.m., Student’s t -test * P <0.05; ** P <0.01; *** P <0.001. Scale bars, 10 μm. 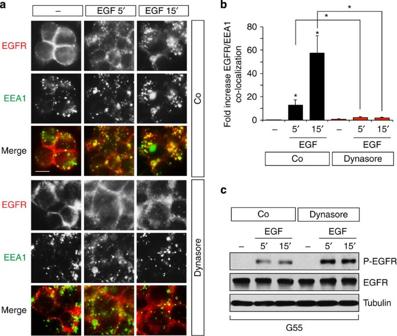Figure 4: Impairment of EGFR internalization phenocopies PHD3 loss. (a,b) Dynasore inhibits EGFR internalization. G55 cells were treated for 2 h with DMSO control or dynasore (0.32 mM), an inhibitor of dynamin-dependent endocytosis. EGFR co-localizes at early time points with EEA1, peaking at 15 min after stimulation. Dynasore compromises EGFR internalization, with EGFR remaining at the plasma membrane (a). Quantification of the increase in EGFR/EEA1 co-localization relative to non-stimulated cells (n=50–200) is shown inb. (c) Impairment of EGFR internalization increases EGFR phosphorylation. Immunoblot of G55 cells non-stimulated or stimulated with 20 ng ml−1EGF and treated with control DMSO or dynasore. Western blot images (c) have been cropped for presentation. Full-size images are presented inSupplementary Fig. 6. All values are means+s.e.m., Student’st-test *P<0.05. Scale bar, 10 μm. Full size image Figure 4: Impairment of EGFR internalization phenocopies PHD3 loss. ( a , b ) Dynasore inhibits EGFR internalization. G55 cells were treated for 2 h with DMSO control or dynasore (0.32 mM), an inhibitor of dynamin-dependent endocytosis. EGFR co-localizes at early time points with EEA1, peaking at 15 min after stimulation. Dynasore compromises EGFR internalization, with EGFR remaining at the plasma membrane ( a ). Quantification of the increase in EGFR/EEA1 co-localization relative to non-stimulated cells ( n =50–200) is shown in b . ( c ) Impairment of EGFR internalization increases EGFR phosphorylation. Immunoblot of G55 cells non-stimulated or stimulated with 20 ng ml −1 EGF and treated with control DMSO or dynasore. Western blot images ( c ) have been cropped for presentation. Full-size images are presented in Supplementary Fig. 6 . All values are means+s.e.m., Student’s t -test * P <0.05. Scale bar, 10 μm. Full size image PHD3 regulates the binding of endocytic adaptors to EGFR To obtain additional mechanistic insight into the function of PHD3 in EGFR internalization and to confirm that PHD3 acts as a scaffolding adaptor that regulates the early steps of EGFR endocytosis, we next analysed the role of PHD3 in the recruitment of known EGFR interactors that play a central part in EGFR internalization and signalling. Binding of the E3 ligase Cbl, in complex with Grb2, to phosphorylated EGFR has been shown to act as a switch that tightly regulates the ubiquitination of the receptor and can trigger its internalization [29] . Therefore, we first investigated whether the recruitment of Cbl and Grb2, as well as the ubiquitination levels of EGFR, were altered following PHD3 loss. In agreement with a disruption of the internalization of EGFR that is consequently maintained at the plasma membrane in a hyperphosphorylated state (see, for example, Figs 1a and 3a–d ), cells lacking PHD3 showed an increased recruitment of c-Cbl, Cbl-b and Grb2, as well as increased levels of receptor ubiquitination ( Fig. 5a,b ). 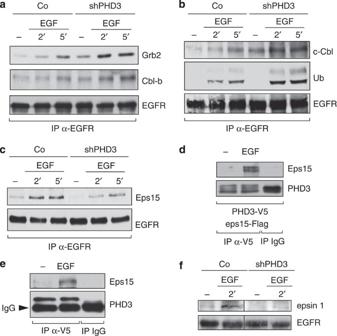Figure 5: PHD3 regulates the recruitment of Eps15 and epsin1 to EGFR. (a,b) PHD3 loss increases Grb2, Cbl-b and c-Cbl recruitment to EGFR, as well as EGFR ubiquitination. Immunoblot of Grb2 and Cbl-b (a) and of c-Cbl and ubiquitin (b) of immunoprecipitated EGFR from G55 cells expressing control or PHD3 shRNA that were non-stimulated or EGF stimulated for the indicated times. (c) Recruitment of the endocytic adaptor Eps15 is impaired following PHD3 loss. Immunoblot of Eps15 of immunoprecipitated EGFR from G55 cells expressing control or PHD3 shRNA that were non-stimulated or EGF stimulated for the indicated times. (d,e) PHD3 and Eps15 interact. Co-immunoprecipitation assay using anti-V5 antibodies or IgG control from extracts of G55 cells expressing PHD3-V5 and Eps15-Flag (d) or PHD3-V5 (e) and western blot of Eps15 and PHD3, demonstrating interaction of PHD3 with exogenous and endogenous Eps15, respectively. Cells were non-stimulated or stimulated with EGF (20 ng ml−1) for 5 min. (f) Recruitment of the endocytic adaptor epsin1 is impaired following PHD3 loss. Immunoblot of epsin1 of immunoprecipitated EGFR from G55 cells expressing control or PHD3 shRNA that were non-stimulated or EGF stimulated for 2 min. Western blot images (a–f) have been cropped for presentation. Full-size images are presented inSupplementary Fig. 7. Figure 5: PHD3 regulates the recruitment of Eps15 and epsin1 to EGFR. ( a , b ) PHD3 loss increases Grb2, Cbl-b and c-Cbl recruitment to EGFR, as well as EGFR ubiquitination. Immunoblot of Grb2 and Cbl-b ( a ) and of c-Cbl and ubiquitin ( b ) of immunoprecipitated EGFR from G55 cells expressing control or PHD3 shRNA that were non-stimulated or EGF stimulated for the indicated times. ( c ) Recruitment of the endocytic adaptor Eps15 is impaired following PHD3 loss. Immunoblot of Eps15 of immunoprecipitated EGFR from G55 cells expressing control or PHD3 shRNA that were non-stimulated or EGF stimulated for the indicated times. ( d , e ) PHD3 and Eps15 interact. Co-immunoprecipitation assay using anti-V5 antibodies or IgG control from extracts of G55 cells expressing PHD3-V5 and Eps15-Flag ( d ) or PHD3-V5 ( e ) and western blot of Eps15 and PHD3, demonstrating interaction of PHD3 with exogenous and endogenous Eps15, respectively. Cells were non-stimulated or stimulated with EGF (20 ng ml −1 ) for 5 min. ( f ) Recruitment of the endocytic adaptor epsin1 is impaired following PHD3 loss. Immunoblot of epsin1 of immunoprecipitated EGFR from G55 cells expressing control or PHD3 shRNA that were non-stimulated or EGF stimulated for 2 min. Western blot images ( a – f ) have been cropped for presentation. Full-size images are presented in Supplementary Fig. 7 . Full size image Despite the increased ubiquitination, which can rapidly trigger EGFR endocytosis, the receptor failed to internalize in PHD3-deficient cells, indicating that PHD3 might be important for the recruitment of downstream components of the EGFR internalization machinery, such as early endocytic adaptors. EGFR pathway substrate (Eps) 15 and epsin1 are members of a family of ubiquitin-interacting motif (UIM) containing proteins that govern the early steps of EGFR endocytosis [30] , [31] , [32] . Therefore, we investigated whether the loss of PHD3 affects the recruitment of Eps15 and epsin1 to EGFR. The recruitment of Eps15 following EGF stimulation was prominently reduced in cells deficient for PHD3 ( Fig. 5c ), indicating that PHD3 acts as a scaffolding protein that directs the recruitment of Eps15 to EGFR. Importantly, and in agreement with this model, PHD3 physically interacted with Eps15 following stimulation with EGF ( Fig. 5d,e ). In addition, PHD3 disruption reduced the recruitment of epsin1 to EGFR ( Fig. 5f ). Collectively, these data suggest a model in which inactivation of PHD3 sustains proliferative signalling and promotes tumour growth by increasing EGFR activity as a result of impaired recruitment of early endocytic adaptor proteins such as Eps15 and epsin1, thereby suppressing EGFR internalization. PHD3 controls EGFR signalling in response to hypoxia We have demonstrated that PHD3 levels are highly upregulated by growth-inhibitory signals, including hypoxia, tumour-necrosis factor-α, hypoglycaemia and growth factor deprivation (see Henze et al. [28] ). Given the importance of PHD3 in growth control, we next addressed whether the increased PHD3 levels could relay growth-inhibitory signals by impairing EGFR signalling. Indeed, exposure of the glioma cell line G141 to hypoxia, which highly induces PHD3 expression, led to a striking reduction of EGFR signalling, whereas PHD3 loss allowed for a continued increased EGFR signalling under hypoxia ( Fig. 6a ). The results indicate that PHD3 mediates growth inhibition through suppression of EGFR activation. To directly confirm that enhanced PHD3 expression leads to inhibition of EGFR signalling, we used G55 cells with increased PHD3 levels, and control G55 cells expressing green fluorescent protein (GFP). Importantly, PHD3 overexpression decreased phosphorylation of EGFR ( Fig. 6b ) and suppressed downstream signalling as evidenced by decreased levels of phosphorylation of MAPK ( Fig. 6c ) and reduced SRE promoter reporter activity ( Supplementary Fig. 4 ). Moreover, analysis of EGFR endocytosis by immunofluorescence demonstrated that the decreased EGFR phosphorylation and signalling following PHD3 overexpression was accompanied by an accelerated rate of receptor internalization ( Fig. 6d,e ), which was blocked by dynasore treatment ( Fig. 6d,e ). Importantly, and in agreement with a crucial role of PHD3 as a scaffold protein recruiting Eps15 to promote EGFR endocytosis, overexpression of PHD3 resulted in an increased recruitment of Eps15 to EGFR ( Fig. 6f ). Collectively, these findings demonstrate that EGFR responses are highly sensitive to PHD3 expression levels, indicating that PHD3 is a crucial regulator and a limiting factor for EGFR function. 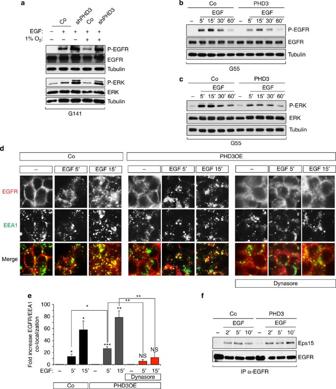Figure 6: Enhanced PHD3 expression inhibits EGFR signalling. (a) PHD3 loss attenuates the hypoxia-mediated inhibition of EGFR signalling. Immunoblot of G141 tumour cells expressing control or PHD3 shRNA, following exposure to 21% (−) or 1% O2(+) for 48 h±EGF (20 ng ml−1) for 5 min. (b,c) EGFR phosphorylation and signalling is attenuated by PHD3. Immunoblot with (P-)EGFR (b) and (P-)ERK (c) of G55 cells expressing PHD3 or GFP control. (d,e) Internalization of EGFR assessed by immunofluorescence in G55 cells expressing PHD3 or GFP control non-stimulated or stimulated with EGF (20 ng ml−1) for the indicated times. The co-localization of EGFR with EEA1 induced by EGF is significantly increased in cells expressing exogenous PHD3 in comparison with the controls. The increased internalization induced by PHD3 overexpression is blocked by dynasore (d). Quantification of the increase in EGFR/EEA1 co-localization relative to non-stimulated cells (n=50–200) is shown ine. (f) Overexpression of PHD3 enhances the recruitment of the endocytic adaptor Eps15 to EGFR. Immunoblot of Eps15 of immunoprecipitated EGFR (IP α-EGFR) from G55 cells expressing PHD3 or GFP control that were non-stimulated or EGF stimulated for the indicated times. Western blot images (a–c,f) have been cropped for presentation. Full-size images are presented inSupplementary Fig. 8. All values are means+s.e.m., Student’st-test *P<0.05; **P<0.01; ***P<0.001. Scale bar, 10 μm. Figure 6: Enhanced PHD3 expression inhibits EGFR signalling. ( a ) PHD3 loss attenuates the hypoxia-mediated inhibition of EGFR signalling. Immunoblot of G141 tumour cells expressing control or PHD3 shRNA, following exposure to 21% (−) or 1% O 2 (+) for 48 h±EGF (20 ng ml −1 ) for 5 min. ( b , c ) EGFR phosphorylation and signalling is attenuated by PHD3. Immunoblot with (P-)EGFR ( b ) and (P-)ERK ( c ) of G55 cells expressing PHD3 or GFP control. ( d , e ) Internalization of EGFR assessed by immunofluorescence in G55 cells expressing PHD3 or GFP control non-stimulated or stimulated with EGF (20 ng ml −1 ) for the indicated times. The co-localization of EGFR with EEA1 induced by EGF is significantly increased in cells expressing exogenous PHD3 in comparison with the controls. The increased internalization induced by PHD3 overexpression is blocked by dynasore ( d ). Quantification of the increase in EGFR/EEA1 co-localization relative to non-stimulated cells ( n =50–200) is shown in e . ( f ) Overexpression of PHD3 enhances the recruitment of the endocytic adaptor Eps15 to EGFR. Immunoblot of Eps15 of immunoprecipitated EGFR (IP α-EGFR) from G55 cells expressing PHD3 or GFP control that were non-stimulated or EGF stimulated for the indicated times. Western blot images ( a – c , f ) have been cropped for presentation. Full-size images are presented in Supplementary Fig. 8 . All values are means+s.e.m., Student’s t -test * P <0.05; ** P <0.01; *** P <0.001. Scale bar, 10 μm. Full size image Here we identify PHD3 as a novel regulator of EGFR signalling that limits EGFR-activated proliferation and survival in response to hypoxia. Our findings support a model for the function of PHD3 in growth control, in which PHD3 acts as a signalling hub that integrates growth-inhibitory and -stimulatory signals to control EGFR activity. Tumour cells with decreased PHD3 levels, for example, as a result of epigenetic silencing or deletion, hyperactivate EGFR signalling by attenuating EGFR internalization and become refractory to growth-inhibitory signals ( Fig. 7 ). Collectively, our data uncover a key mechanism through which tumour cells attain central hallmarks of cancer by PHD3 inactivation. 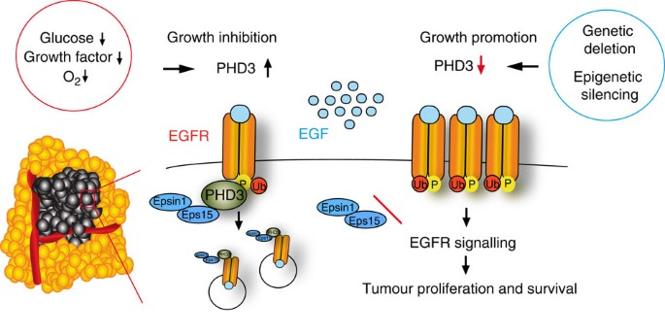Figure 7: Model of PHD3 function in the control of tumour growth. PHD3 is induced by hypoxia to promote the recruitment of Eps15 and epsin1 and promote EGFR internalization, which leads to attenuation of EGFR signalling and function. Silencing of PHD3 expression during tumour progression (for example, by genetic deletion or epigenetic silencing) impairs Eps15 and epsin1 recruitment and EGFR internalization. As a consequence, EGFR is retained at the membrane, resulting in the acquisition of growth signal autonomy through hyperactivation of EGFR and thus increasing tumour resistance to the growth-inhibitory and pro-apoptotic effects of hypoxia. Figure 7: Model of PHD3 function in the control of tumour growth. PHD3 is induced by hypoxia to promote the recruitment of Eps15 and epsin1 and promote EGFR internalization, which leads to attenuation of EGFR signalling and function. Silencing of PHD3 expression during tumour progression (for example, by genetic deletion or epigenetic silencing) impairs Eps15 and epsin1 recruitment and EGFR internalization. As a consequence, EGFR is retained at the membrane, resulting in the acquisition of growth signal autonomy through hyperactivation of EGFR and thus increasing tumour resistance to the growth-inhibitory and pro-apoptotic effects of hypoxia. Full size image Several studies have highlighted the importance of EGFR internalization by endocytosis for the regulation of EGFR activity, as well as the role of the oxygen-sensing pathway in this process [5] , [33] . Our findings uncover a novel role for PHD3 as a scaffolding protein that mediates the recruitment of early endocytic adaptors such as Eps15 and epsin1 to EGFR. This function of PHD3 is separate from the HIF-, nuclear factor-κB and hydroxylation-dependent functions of PHD3. Eps15 is an essential component of the EGFR internalization machinery that acts in concert with epsin1 (ref. 34 ). The essential requirement of Eps15 and epsin1 for EGFR internalization is underlined by several studies. Inhibition of Eps15 function by RNA interference (RNAi) [35] , [36] , [37] , microinjection of neutralizing antibodies [38] or a dominant-negative mutant [39] , as well as epsin1 inhibition [40] have been shown to significantly reduce EGFR internalization. Therefore, impaired recruitment of Esp15 and epsin1 may fully explain the effect of PHD3 loss on EGFR endocytosis and signalling. However, our data do not preclude the possibility that PHD3 might regulate the binding of additional UIM-containing components of the endocytic machinery besides Eps15 and epsin1, which are involved in EGFR endocytosis [31] . Eps15 and espin1 interact with ubiquitinated cargos through their UIM [30] . Despite the increased ubiquitination of EGFR, Eps15 failed to be efficiently recruited to EGFR in the absence of PHD3. These data suggest that either the scaffolding function of PHD3 may be important for the UIM mediated interaction of Eps15 with EGFR or that PHD3 promotes binding of Eps15 to EGFR in a manner independent of EGFR ubiquitination and the UIM of Eps15. In fact, Eps15 is known to bind to EGFR in an UIM-independent manner through its central coiled-coil domain [41] . It will be interesting to study further how and through which domains PHD3 affects the UIM-dependent and -independent binding of endocytic proteins to EGFR in such a cooperative model. Collectively, our work identifies the impairment of PHD3-mediated EGFR internalization as a novel mechanism through which tumour cells induce deregulation of EGFR activity to sustain proliferative signalling even at low oxygen tension. A number of recent reports suggest that the regulation of receptor activity and trafficking is a more general function of PHD3. PHD3 is involved in the regulation of the trafficking and activity of the β2-adrenergic receptor [17] and the TRPA1 ion channel [42] ; moreover, the Caenorhabditis elegans PHD homologue, Egl-9E, has been recently shown to regulate the trafficking of glutamate receptor 1 to the plasma membrane [43] . It is therefore tempting to speculate that the regulation of receptor trafficking may be an important function of PHD3 to flexibly respond to microenvironmental cues. Our findings of a PHD3-dependent regulation of EGFR internalization add a prominent example to a growing body of evidence that highlights the importance of receptor endocytosis in cancer progression [44] . Together with the accompanying paper by Henze et al. [28] , we demonstrate that PHD3 acts as a central mediator of hypoxia and possibly other growth-inhibitory signals by suppressing EGFR signalling, whose silencing by genetic or epigenetic mechanisms may serve as an alternative mechanism to activate EGFR and potentiate tumour growth. Thus, our findings highlight the importance of the PHD3-dependent control of EGFR signalling in tumour biology, revealing novel mechanisms that regulate tumour growth and progression. Cell culture The glioblastoma cell lines G55TL and G141 were kindly provided by M. Westphal and K. Lamszus (Hamburg, Germany) and HGBM by H. Weich (Braunschweig, Germany). Glioblastoma cell lines were cultured in DMEM (Invitrogen) supplemented with 10% fetal bovine serum (PAN Systems). For propagating cells under neurosphere conditions, cell culture dishes, plates or flasks were coated with 10 mg ml −1 poly(2-hydroxyethyl methacrylate) (pHEMA) and dried. Neurosphere medium (DMEM-F12 (Gibco, Invitrogen, Carlsbad, CA), 2% B-27 Serum-Free Supplement (Invitrogen, Carlsbad, CA)) was supplemented with 20 ng ml −1 basic fibroblast growth factor (bFGF) and 20 ng ml −1 epidermal growth factor (EGF) (PeproTech, Hamburg, Germany). The primary glioblastoma line GBM046x was obtained from a patient undergoing surgery in accordance with a protocol approved by the institutional review board and cultured in neurosphere medium. Following lentiviral transduction, cells were cultured with 2–6 μg ml −1 blasticidin or 2 μg ml −1 puromycin depending on the respective vector system. The PHD3 −/− and control murine astrocytomas were generated as described [28] . All cells were maintained at 37 °C in 5% CO 2 . For overexpression, G55TL cells were stably transfected with the pTet-Off regulator plasmid (Clontech) and the pTRE2hyg/pur-PHD2, -PHD3 or -GFP-inducible expression plasmids and selected with 200 μg ml −1 hygromycin. For hypoxic treatment, cells were grown at 1% O 2 for the indicated time points in a Hypoxic Workstation (Ruskinn Technology, Pencoed, UK; Coy Lab, Grass Lake, USA). Reagents The following reagents were used: 10 μM MEK1 and MEK2 inhibitor U0126 (InvivoGen) and 0.32 mM dynasore (Sigma-Aldrich). Plasmids/small interfering RNA pTet-Off was purchased from BD Bioscience Clontech. PHD2, PHD3 and GFP complementary DNA were subcloned into the pTRE2hyg/pur vector (BD Bioscience Clontech) to generate the pTRE2hyg/pur-PHD3 or -GFP-inducible expression plasmids. The PHD3 expression plasmids HA-EGLN3 wt-pcDNA3 and HA-EGLN3 H196A-pcDNA3 were a kind gift from W. Kaelin (Boston, USA) [27] . Empty control vector pcDNA3 was purchased from Invitrogen and pGIPZ lentiviral shRNAmir vectors for HIF-1α, HIF-2α and pGIPZ non-silencing control were purchased from Open Biosystems. The Block-it Pol II miR RNAi Expression Vector Kit (Invitrogen) was used to construct pcDNA6.2-GW/EmGFP-miR vectors (Invitrogen) expressing the target (PHD3 and PHD2) miRNAs (shRNAs) according to the manufacturer’s instructions using specific miRNA sequences ( Supplementary Table 1 ); miRNA/shRNA targeting the Drosophila SIMA gene was used as control. The rapid attB and attP sites (BP)/attL and attR sites (LR) recombination reaction (Block-it Lentiviral Pol II miR RNAi Expression System, Invitrogen) between pDONR 221, pcDNA6.2-GW/EmGFP-miR and pLenti6/V5-DEST was performed to generate the pLenti6/V5-GW/EmGFP-miR expression construct. The MAPK constitutive active construct ERK2-MEK1 was a kind gift of B. Brüne (Frankfurt, Germany) [45] and the pMT2.SM Flag-Eps15 plasmid was a kind gift of J. Borst (NKI, The Netherlands) [46] . All plasmids were confirmed by DNA sequencing. Small interfering RNA (siRNA) against EGFR was obtained as a pool of four siRNA oligos (Dharmacon ON-TARGETplus SMARTpool siRNAs, Thermo Scientific). Transfection, virus production and infection G55TL cells were stably transfected with the pTet-Off regulator plasmid (Clontech) and the pTRE2hyg/pur-PHD3 or -GFP-inducible expression plasmids, selected with 200 μg ml −1 hygromycin and screened for low transgene background and high transgene induction by western blot and quantitative PCR analysis. Lentiviral particles with the pGIPZ vectors were produced according to the manufacturer’s instructions using the Trans-Lentiviral shRNA Bulk Packaging System (Open Biosystems). Cells were selected with 2 μg ml −1 puromycin to obtain resistant polyclonal cell pools. Lentiviral particles were produced in HEK293T cells using the ViraPower Lentiviral Expression System (Invitrogen) and Lipofectamine 2000 according to the manufacturer’s instructions or the pCI-VSVG and psPAX2 packaging plasmids and calcium phosphate transfection. G55TL and HGBM were selected with 6 μg ml −1 and G141 with 4 μg ml −1 puromycin to obtain resistant polyclonal cell pools. Gene expression analysis was performed using western blot and quantitative PCR. Sphere-forming units and in vitro growth For quantification of sphere-forming units, cells were seeded at 500–1,000 cells per well in pHEMA (10 mg ml −1 pHEMA in 95% ethanol)-coated six-well suspension culture plates ( n =6). The cells were incubated in Neurosphere medium (see above)±the addition of growth factors and, where applicable, respective reagents. Ninety-six hours later, the spheres were counted and the percentage of sphere-forming cells was calculated. Immunofluorescence Cells (200,000) were seeded on pHEMA-coated 6-cm dishes and cultivated as tumour spheres in medium devoid of growth factors for 48 h±5 min of EGF stimulation. Spheres were transferred onto a slide using a Cyto-Tek Centrifuge (Sakura Finetek). Fixation was performed in 4% paraformaldehyde (PFA) for 10 min at 4 °C followed by a rinse in PBS (two times 2 min). Blocking solution was applied (PBS/0.1% Triton X-100/1% BSA/4% donkey serum) for 30 min followed by incubation with rabbit anti-EGFR antibody (1:200 in blocking solution, Cell Signalling), mouse monoclonal EEA1 antibody (1:200 in blocking solution, BD Biosciences) or mouse monoclonal M6PR antibody (1:100 in blocking solution, Abcam) for 1 h at room temperature (RT). Slides were washed three times with PBS/0.1% Triton X-100 and incubated with secondary anti-rabbit Cy3 and anti-mouse Alexa 488 antibodies (diluted 1:200 in blocking solution) for 1 h at RT. Cells were washed three times with PBS, once with water and mounted using VECTASHIELD mounting medium (Vector Laboratories). For quantification of EGFR internalization in early and late endosomes, the fraction of cell area in which EGFR co-localized with EEA1 or M6PR signals, respectively, was measured and normalized to the co-localization area without EGF treatment. The software Metamorph was used to analyse the co-localization of signals from the EAA1 or M6PR and the EGFR channels. On average, the areas of co-localization were analysed in 50–200 cells for these experiments. The fraction of cell area in which EGFR co-localized with EEA1 or M6PR signals, respectively, was measured and normalized to the co-localization area without EGF treatment. The graph represents the fold of increased co-localization with respect to the value in non-stimulated conditions, which in every case is set to 1. Throughout the manuscript, the values were always internally normalized for one cell type (control, shPHD3, wild-type astrocytomas, PHD3KO astrocytomas, PHD3-overexpressing cells) to its own non-stimulated controls. For PHD3 co-staining, the spheres were permeabilized for 4 min on ice with 0.1% Triton X-100 in PBS and washed with PBS. The blocking solution (PBS/2% BSA/4% donkey serum) was applied for 30 min. Subsequently, the spheres were incubated with rabbit anti-EGFR (1:200 in blocking solution, Cell Signalling), goat anti-PHD3 (1:200 in blocking solution, Santa Cruz) and mouse anti-EEA1 (1:200 in blocking solution, BD Biosciences) for 90 min at RT. After intensive washing with PBS, the slides were incubated with secondary anti-rabbit Alexa 488, anti-goat Cy3 and anti-mouse Cy5 (all diluted, 1:200 in blocking solution) for 1 h at RT. Slides were washed three times with PBS, once with water and mounted using DAKO mounting medium. Surface EGFR FACS G55TL cells were seeded at 500,000 cells per 10 cm pHEMA-coated dish in triplets and incubated for 24 h in F12 medium without EGF/FGF. After treatment with EGF for the indicated times, the spheres were immediately fixed in ice-cold 1% PFA for 30 min at 4 °C. After extensive washing with FACS staining buffer (PBS, pH 7.2, 0.5% BSA, 2 mM EDTA), the spheres were dissociated into single cell suspension by treatment with accutase containing 100 U ml −1 DNAse I (Sigma-Aldrich) for 15 min at 37 °C. Single cells were separated using a 40-μm cell strainer (BD Falcon). Following two washing steps, the cells were blocked with 20 μl of normal rat IgG (Invitrogen) for 20 min at 4 °C and stained with 5 μl of EGFR-APC-conjugated antibody (#FAB10951A, R&D) for 30 min at 4 °C. The background staining was determined using matching isotype control antibody from the same manufacturer at the same concentration as the specific antibody. Flow cytometry was performed using BD FACS Canto II (BD Biosciences). Data analysis to quantify changes in the mean surface receptor fluorescence values was performed using FlowJo v7/9 (Tree Star). The singlets were gated using forward scatter area versus width and side scatter area versus width. To calculate percent internalization, the mean fluorescence intensity (MFI) of the cells for each data set minus MFI of the cells stained with the matching isotype control antibody was used. The relative percentage of residual cell surface EGFR at each time point was normalized relative to the MFI of the non-stimulated G55TL control cells. Luciferase reporter assay Cells were transiently transfected with an SRE promoter firefly and a SV40-Renilla luciferase construct (Promega) for normalization of transfection efficiency, grown for 48 h under sphere conditions±the addition of the indicated concentrations of EGF (10–20 ng ml −1 ) for the respective times and assayed for luciferase activity with the Dual-Luciferase Reporter-Assay System (Promega). Immunoblotting and immunoprecipitation For immunoblotting, cells were harvested in PBS (4 °C) and cell pellets were lysed in 10 mM Tris/HCl (pH 7.5), 2% SDS, 2 mM EGTA and 20 mM NaF or in 50 mM Tris/HCl buffer (pH 7.5), 1% Triton X-100, 150 mM NaCl, 10 mM sodium pyrophosphate, 20 mM NaF, 1 mM sodium orthovanadate and 1% complete protease inhibitor cocktail (Roche). Protein lysates (25 μg) were subjected to SDS–PAGE and western blot analysis was performed using antibodies specific to PHD3 (Novus Biologicals NB-100-303), V5 (Invitrogen, R960-25), pEGFR (Tyr 1173; Santa Cruz Biotechnology, sc-12351), pEGFR (Tyr 1068; Cell Signalling, #3777), EGFR (Cell Signalling #4267 or Millipore #06-847), pERK (E-4; Santa Cruz Biotechnology, sc-7383), pERK1/2 (Thr202/Thr204; Cell Signalling), ERK2 (c-14; Santa Cruz Biotechnology, sc-154), ERK1/2 (Cell Signalling), Grb2 (1:1,000, BD, #610111), c-Cbl (1:1,000, BD, #610442), Cbl-b (1:500, Santa Cruz Biotechnology, sc-1435), ubiquitin (1:500, Santa Cruz Biotechnology, sc-8017), Eps15 (1:500, Santa Cruz Biotechnology, sc-534), epsin1 (1:1,000, Santa Cruz Biotechnology, sc-55556) and tubulin (Jackson Lab, DLN09992 or Invitrogen) or actin (Santa Cruz Biotechnology, sc-1615) as loading controls. Immunoreactive bands were detected with horseradish peroxidase-conjugated secondary antibodies through enhanced chemiluminescence (Thermo, PerkinElmer and GE Healthcare). For immunoprecipitation, cells were lysed using immunoprecipitation (IP) lysis buffer (50 mM Tris-HCl, pH 7.5, 150 mM NaCl, 0.5% Triton X-100, 10% glycerol, 1 mM sodium orthovanadate (Na 3 VO 4 ), 10 mM NaPPi, 20 mM NaF, protease inhibitors 100 μM p -APMSF hydrochloride (Calbiochem) and complete protease inhibitor cocktail (Roche)) and lysates were clarified by centrifugation at 13,000 g . Immunosorb A beads (25 μl; AB Medicago) were washed three times with phosphate lysis buffer and incubated with 1–2 mg of protein lysate and 1–2 μg of antibody. Control lysate was mixed with normal mouse IgG or normal rabbit IgG and beads. After overnight incubation of antibodies, beads and lysate at 4 °C with rotation, immunoprecipitates were washed three times with 1 ml IP lysis buffer at 4 °C. 2 × loading buffer was added and samples were boiled at 95 °C for 5 min, spun to pellet the beads and subjected to SDS–PAGE (immunoprecipitate or 35 μg of total lysate). For phosphotyrosine immunoprecipitation, cells were lysed in 20 mM Tris-HCl, pH 7.5, 137 mM NaCl, 1 mM MgCl 2 , 0.1 mM CaCl 2 , 1 mM Na 3 VO 4 , 1 mM phenylmethylsulfonyl fluoride (PMSF), 10% glycerol, 10 μg of leupeptin ml −1 and 5 μg of aprotinin ml −1 . Agarose G beads and anti-phosphotyrosine antibody (4G10, Millipore) were added directly to the cell lysate at a final concentration of 2 μg of antibody per 300 μg of protein. The samples were rotated end-over-end for 4 h at 4 °C, and the immune complexes were collected by centrifugation in a microcentrifuge. The immunoprecipitated proteins were released by boiling for 5 min at 95 °C in SDS–PAGE sample buffer. The agarose beads were removed by centrifugation before loading the samples on 8% SDS–PAGE gel. For EGFR immunoprecipitation, G55 cells grown in neurosphere conditions that were unstimulated or stimulated with 20 ng ml −1 EGF for the indicated times were lysed in NP-40 buffer (50 mM Tris, pH 7.4, 1% NP-40, 150 mM NaCl, 4 mM EDTA and 5% glycerol) with phosphatase and protease inhibitors. Lysates were incubated with EGFR antibody (Santa Cruz Biotechnology, #sc-120) overnight at 4 °C with continuous mixing. Immunoprecipitated material was washed four times with NP-40 buffer and boiled in SDS buffer. To analyse the interaction between PHD3 and Eps15, PHD3-V5-overexpressing G55 cells were cultured in neurosphere conditions, were lysed and immunoprecipitated with V5 antibody (Invitrogen, #R960-25) as described earlier. All representative western blots included in the manuscript are shown as full scans in Supplementary Figs 5–9 . Internalization assay and capture ELISA PHD3 knockout or control murine astrocytoma cells (600,000) were plated in pHEMA-coated 10-cm dishes and cultured for 4 days under sphere conditions. Spheres were collected, placed on ice and washed in HBSS with Ca 2+ and Mg 2+ . To label surface proteins, spheres were incubated with 0.5 mg ml −1 EZ-Link-NHS-SS-Biotin (Thermo Scientific) in HBSS with Ca 2+ and Mg 2+ for 15 min at 4 °C with rotation. Excessive biotin was quenched with 5 mM Tris-HCl (pH 7.5) in HBSS with Ca 2+ and Mg 2+ , the spheres were stimulated with 20 ng ml −1 EGF diluted in HBSS with Ca 2+ and Mg 2+ for 2–60 min at 37 °C (as indicated). Surface-remaining biotin was cleaved with 150 mM reduced L -glutathione in 150 mM NaCl for 25 min on ice. After extensive washing with HBSS with Ca 2+ and Mg 2+ , spheres were lysed in 50 mM Tris/HCl buffer (pH 7.5), 1% Triton X-100, 150 mM NaCl, 10 mM sodium pyrophosphate, 20 mM NaF, 1 mM sodium orthovanadate and 1% complete protease inhibitor cocktail (Roche). Ninety-six-well Maxisorp plates (Nunc) were pre-coated with 2 μg ml −1 mouse anti-EGFR (monoclonal, Santa Cruz Biotechnology) overnight at 4 °C. The pre-coated ELISA plates were washed with 0.01% Tween-20 in PBS and blocked with 5% fetal bovine serum (FBS) in PBS for 2 h at RT. Subsequently, the plates were washed again with 0.01% Tween-20 in PBS and lysates with equal amounts of protein were added to the plate overnight at 4 °C. The ELISA plates were washed and streptavidin-horseradish peroxidase (1:2,000, R&D systems) diluted in 1% FBS–PBS was applied for 30 min at RT. After extensive washing, the substrate reagent solution (tetramethylbenzidine, R&D systems) was added for detection of biotinylated EGFR bound to the ELISA plate. The colour reaction was stopped with 2N sulfuric acid (R&D systems), and the plate read at 450 nm. As a control, lysates with equal amounts of protein were in parallel added to wells without mouse anti-EGFR. This background signal was subtracted from the samples; samples with a signal level below background were set to 0. The rate of internalization was calculated as the fold increase of internalized receptor following stimulation with EGF in comparison with the non-stimulated sample. The rate of internalization was calculated for each cell type individually, normalizing to its own non-stimulated sample. Proximity ligation assay Cells were dissociated with accutase counted and fixed with 4% PFA in PBS for 10 min. The cells were then transferred onto glass slides using a Cyto-Tek Centrifuge (Sakura Finetek). The cells were permeabilized using 0.1% Triton X-100 in PBS for 4 min on ice. Subsequently, the cells were washed with PBS and blocking solution (2% BSA, 4% donkey serum in PBS) was applied for 30 min at 37 °C in a humidified chamber. The primary antibodies against EGFR (mouse monoclonal, 1:400, Santa Cruz Biotechnology) and PHD3 (rabbit polyclonal, 1:400, Novus Biologicals) diluted in blocking solution were added for 30 min at 37 °C. The cells were then washed with buffer A of the Duolink II proximity ligation assay kit according to the manufacturer’s instructions (Olink Bioscience). Subsequently, the Duolink II PLA probe anti-mouse Minus and the Duolink II PLA probe anti-rabbit Plus together with phalloidin-fluorescein isothiocyanate (1:250) were added to the cells for 60 min at 37 °C. Following another washing step in buffer A, the cells were incubated in the Duolink II ligation buffer diluted in distilled water with ligase for 30 min at 37 °C to link the two probes by enzymatic ligation. Subsequently, the cells were washed in buffer A, and the Duolink II orange amplification buffer diluted in distilled water together with the polymerase was applied to the cells for 100 min at 37 °C. After the amplification step, the cells were washed several times in buffer B of the Duolink II proximity ligation assay kit. During one of the washing steps, 4',6-diamidino-2-phenylindole (1:1,000) diluted in wash buffer B was added. Finally, the cells were mounted using the Antifade Kit (Invitrogen). Statistical analysis Results are presented as mean±s.e.m. Statistical analysis was performed using the Student’s t -test. Statistical significance was defined as P <0.05 (* P <0.05; ** P <0.01; *** P <0.001). How to cite this article: Garvalov, B. K. et al. PHD3 regulates EGFR internalization and signalling in tumours. Nat. Commun. 5:5577 doi: 10.1038/ncomms6577 (2014).